Formation of nickel cobalt sulfide ball-in-ball hollow spheres with enhanced electrochemical pseudocapacitive properties While the synthesis of hollow structures of transition metal oxides is well established, it is extremely challenging to fabricate complex hollow structures for mixed transition metal sulfides. Here we report an anion exchange method to synthesize a complex ternary metal sulfides hollow structure, namely nickel cobalt sulfide ball-in-ball hollow spheres. Uniform nickel cobalt glycerate solid spheres are first synthesized as the precursor and subsequently chemically transformed into nickel cobalt sulfide ball-in-ball hollow spheres. When used as electrode materials for electrochemical capacitors, these nickel cobalt sulfide hollow spheres deliver a specific capacitance of 1,036 F g −1 at a current density of 1.0 A g −1 . An asymmetric supercapacitor based on these ball-in-ball structures shows long-term cycling performance with a high energy density of 42.3 Wh kg −1 at a power density of 476 W kg −1 , suggesting their potential application in high-performance electrochemical capacitors. Owing to their unique structural features and intriguing properties, hollow micro-/nanostructures with tunable size, shape, composition and interior architecture have attracted growing research interests for various applications, such as energy storage, catalysis, chemical sensors and biomedicine [1] , [2] , [3] , [4] , [5] , [6] , [7] , [8] . In the past decade, different types of hollow structures including hollow spheres [9] , [10] , [11] , [12] , boxes [13] , [14] , [15] , [16] and micro-/nanotubes [17] , [18] , [19] have been successfully synthesized through different synthesis routes. However, the configuration of most of available hollow structures appears relatively simple, such as single-shelled hollow spheres of one composition. Recently, extensive research efforts have been devoted to design and fabricate complex hollow structures with multi-shelled architecture and tunable chemical composition, which are expected to realize their optimized physical/chemical properties for specific applications. Until now, many types of metal oxides with multi-shelled structures have been successfully fabricated based on soft- or hard-template methods [20] , [21] , [22] , [23] , [24] , [25] . For example, Lou et al . [26] , [27] have previously fabricated double-shelled SnO 2 hollow spheres using silica spheres as templates combining with designed procedures. Multi-shelled Cu 2 O hollow spheres have also been prepared using cetyl trimethylammonium bromide as soft template [28] . Wang et al . [29] synthesized multi-shelled Co 3 O 4 hollow microspheres with carbonaceous microspheres as hard templates, which exhibit higher lithium storage capacity and improved cycling performance compared with single-shelled Co 3 O 4 microspheres. Very recently, we have developed a new ‘penetration–solidification–annealing’ method to synthesize various mixed metal oxide multi-shelled hollow spheres [30] . Despite these exciting advances, present studies on complex hollow structures are generally limited to metal oxides. Recently, transition metal sulfides have attracted great attention because of their excellent properties and promising applications in electronic, optical and optoelectronic devices [31] , [32] , [33] , [34] , [35] . In particular, ternary nickel cobalt sulfides have been regarded as a promising class of electrode materials for high-performance energy storage devices, since they offer higher electrochemical activity and higher capacity than mono-metal sulfides [36] , [37] , [38] , [39] . Moreover, nickel cobalt sulfides might exhibit much higher conductivity than corresponding ternary nickel cobalt oxides due to the smaller band gap [40] , [41] . Transition metal sulfides hollow structures reported so far with high quality usually possess simple configurations. It is very challenging to synthesize complex hollow structures of metal sulfides on the basis of protocols established for metal oxides because of the distinct physical/chemical properties between these two types of materials. Herein we report a facile anion exchange method to synthesize a novel ball-in-ball hollow structure of ternary nickel cobalt sulfide (NiCo 2 S 4 ). The synthesis involves a facile solvothermal synthesis of metal-glycerate solid spheres and subsequent sulfidation in the presence of thioacetamide (TAA) to form NiCo 2 S 4 ball-in-ball hollow spheres. Importantly, the interiors of the as-prepared NiCo 2 S 4 hollow spheres can be easily tuned by varying the reaction temperature during the anion exchange process. When used as electrode materials for electrochemical capacitors, the NiCo 2 S 4 ball-in-ball hollow spheres deliver excellent pseudocapacitve performance with high specific capacitance and remarkable rate capability. Formation of ball-in-ball hollow spheres We first develop a facile solvothermal method to prepare uniform nickel cobalt glycerate (NiCo-glycerate) spheres as the precursor (see Method for detailed synthesis procedure). Only a broad diffraction peak at around 12° can be seen in the X-ray diffraction (XRD) pattern of NiCo-glycerate ( Supplementary Fig. 1 ), which is a characteristic of metal alkoxides [42] . The NiCo-glycerate spheres are highly uniform with a diameter of around 550 nm ( Supplementary Fig. 2a ). The size distribution can be controlled by adjusting the solvothermal reaction temperature ( Supplementary Fig. 3 ). A solution sulfidation process under solvothermal condition is then utilized to convert the NiCo-glycerate solid precursors into ball-in-ball NiCo 2 S 4 hollow spheres. The whole formation process can be generally divided into three stages as schematically illustrated in Fig. 1 . At stage I, sulfide (S 2− ) ions released from the decomposition of TAA at high temperature react with metal ions on the surface of NiCo-glycerate and produce NiCo-glycerate@NiCo 2 S 4 core–shell structure. This sulfidation process can be described as an anion exchange reaction of the NiCo-glycerate. Further reaction between the inward diffused S 2− ions and faster outward diffused metal cations supplies the growth of the NiCo 2 S 4 shell and leads to a well-defined gap between the shell and the NiCo-glycerate core. When the reaction proceeds to certain degree, it will be more difficult for the metal cations to diffuse to the outer shell through the enlarged empty gap. Thus, a secondary NiCo 2 S 4 shell would be formed on the remaining core as shown at stage II. On the completion of the anion exchange reaction, unique NiCo 2 S 4 ball-in-ball hollow spheres are obtained at the end of stage III. 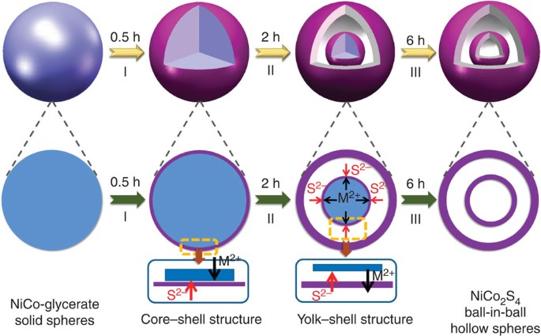Figure 1: Schematic illustration of the formation process of NiCo2S4ball-in-ball hollow spheres. Stage I, surface NiCo2S4formed by anion exchange method. Stage II, further diffusion of S2−and formation of NiCo2S4on the inner NiCo-glycerate core. Stage III, completion of the anion exchange reaction. M2+refers to metal cations including Ni2+and Co2+ions. Figure 1: Schematic illustration of the formation process of NiCo 2 S 4 ball-in-ball hollow spheres. Stage I, surface NiCo 2 S 4 formed by anion exchange method. Stage II, further diffusion of S 2− and formation of NiCo 2 S 4 on the inner NiCo-glycerate core. Stage III, completion of the anion exchange reaction. M 2+ refers to metal cations including Ni 2+ and Co 2+ ions. Full size image To illustrate the formation mechanism of these novel metal sulfide nanostructures, investigations using field-emission scanning electron microscopy (FESEM), transmission electron microscopy (TEM) and powder XRD are conducted to monitor the morphological evolution and crystallization process as a function of the sulfidation time. It can be seen from Fig. 2a,e,i that the NiCo-glycerate precursor is composed of uniform solid spheres without visible pores. The surface of the spheres is very smooth. After sulfidation treatment at 160 °C for 0.5 h, the colour of the obtained product changes from initial brown to black, indicating the formation of metal sulfide. As shown in Fig. 2b,f,j and Supplementary Fig. 2b , the products are still solid spheres but exhibit much rougher surface, which suggests the occurrence of sulfidation reaction on the surface. The surface of these solid microspheres is composed of closely packed nanoparticles. The corresponding XRD pattern demonstrates that these spheres are still mainly NiCo-glycerate with some diminishment in the peak intensity ( Supplementary Fig. 4a ). No diffraction peaks corresponding to NiCo 2 S 4 are found in the XRD pattern, most likely due to its low content and poor crystallinity. When prolonging the sulfidation duration to 2 h, there is an obvious gap between a well-defined shell and a solid core, forming a unique core–shell nanostructure ( Fig. 2g,k ). Such a core–shell nanostructure possesses a porous shell consisting of NiCo 2 S 4 , while retaining a dense core of NiCo-glycerate. The corresponding FESEM images ( Fig. 2c ; Supplementary Fig. 2c ) clearly show that the roughness of the surface increases and some hollow spheres are broken. Two obvious diffraction peaks at 31.5° and 55.3° appear in the corresponding XRD pattern ( Supplementary Fig. 4b ), which can be indexed to the (311) and (440) planes of NiCo 2 S 4 , respectively. Meanwhile, the characteristic peak of NiCo-glycerate at low angle disappears, indicating a gradual phase transformation from NiCo-glycerate to NiCo 2 S 4 . The transformation from solid sphere to core–shell structure is likely due to the discrepancy in diffusion rate between metal cations and sulfide anions during the sulfidation process. However, similar sulfidation reaction generally results in simple hollow structures with a single shell and a completely void interior according to literature reports [17] , [18] , [37] , [38] , [43] . In our work, when further increasing the reaction time to 6 h to complete the reaction, unique ball-in-ball hollow spheres are successfully obtained ( Fig. 2d,h,l ). The roughness of the surface further increases and more visible pores are observed in the shell. At the same time, more broken hollow spheres can be seen from the product ( Supplementary Fig. 2d ). These results imply the growth of primary NiCo 2 S 4 nanoparticles and the slight decrease of mechanical strength of the NiCo 2 S 4 shell. Nevertheless, majority of the NiCo 2 S 4 hollow spheres remain intact and complete, showing satisfactory structural robustness. The corresponding XRD pattern reveals that the NiCo-glycerate precursor is completely transformed into the NiCo 2 S 4 phase ( Supplementary Fig. 4c ). The formation of such novel ball-in-ball hollow structures might be explained by the repeated anion exchange process taking place on the pre-formed solid cores as discussed earlier. 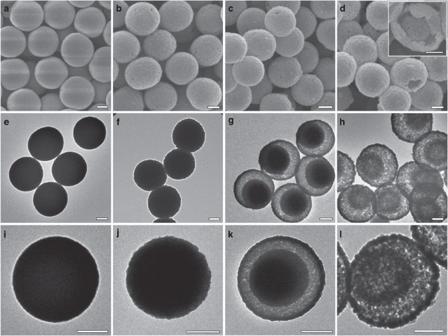Figure 2: FESEM and TEM images of samples. (a,e,i) NiCo-glycerate solid spheres and products obtained after sulfidation of NiCo-glycerate solid spheres at 160 °C for different durations: (b,f,j) 0.5 h; (c,g,k) 2 h; (d,h,l) 6 h. Scale bars, 200 nm. Figure 2: FESEM and TEM images of samples. ( a , e , i ) NiCo-glycerate solid spheres and products obtained after sulfidation of NiCo-glycerate solid spheres at 160 °C for different durations: ( b , f , j ) 0.5 h; ( c , g , k ) 2 h; ( d , h , l ) 6 h. Scale bars, 200 nm. Full size image Controlling the shell structure of hollow spheres One of the crucial factors in the above formation of ball-in-ball hollow spheres is long-lasting supply of sulfide ions from the decomposition of TAA. The spheres obtained after sulfidation at low concentration of TAA are core–shell structures with the inner core diameter of about 400 nm ( Supplementary Fig. 5a ). Ball-in-ball hollow spheres can still be obtained after sulfidation at high concentration of TAA ( Supplementary Fig. 5b ), but the diameter of inner core decreases to only 200 nm. Apart from the concentration of TAA, reaction temperature is another important factor for the formation of hollow spheres, which not only affects the decomposition rate of TAA, but also influences the diffusion rate of ionic species. For example, only core–shell structure is obtained after sulfidation at a lower temperature of 120 °C for 6 h ( Supplementary Fig. 6a,b ). After prolonging the solvothermal reaction to 12 h, similar ball-in-ball hollow spheres can be successfully prepared but with a less pronounced gap between the two layers of shells ( Supplementary Fig. 6c ). Estimated from TEM image ( Supplementary Fig. 6d ), the average diameters of the outer and inner shells are about 590 and 250 nm, respectively. At a lower reaction temperature, the sulfidation process substantially slows down. Moreover, the slower diffusion rate of ionic species especially metal cations results in the formation of the second metal sulfide shell closer to the outer shell. On the contrary, the solid NiCo-glycerate spheres are eventually transformed into NiCo 2 S 4 hollow spheres with the single shell after sulfidation at 200 °C for 6 h ( Supplementary Fig. 7a,b ), as a result of the fast diffusion and anion exchange reaction before the formation of the inner metal sulfide layer on the remaining interior core. These observations also support the formation mechanism of the unique ball-in-ball structure as we discussed earlier. Characterizations of ball-in-ball hollow spheres An annealing treatment at 300 °C in nitrogen (N 2 ) atmosphere is utilized to improve the crystallinity of NiCo 2 S 4 ball-in-ball hollow spheres. From the XRD pattern ( Fig. 3a ), all Bragg peaks can be indexed to cubic NiCo 2 S 4 phase (JCPDS card No. 43–1477). No residues or impurity phases are detected, indicating that the NiCo-glycerate precursor is completely converted to the NiCo 2 S 4 phase after sulfidation. According to the Scherrer formula, the average crystallite size is calculated to be ~14.6 nm, which is consistent with TEM observations. The low-magnification FESEM examination reveals that the NiCo 2 S 4 hollow spheres are still quite uniform, with a diameter of around 600 nm ( Fig. 3b ). An enlarge FESEM image ( Fig. 3c ) shows that the surface of the spheres is very rough, which consists of small nanoparticles. TEM images provide an intuitive way to investigate the interior structure of the spheres by showing notable contrast difference between the hollow and solid parts. TEM images ( Fig. 3d,e ) show that these porous NiCo 2 S 4 spheres exhibit a unique ball-in-ball hollow architecture, which possesses good structural stability to withstand the thermal annealing process. Estimated from TEM images, the average diameters of the outer and inner shells are about 600 and 300 nm, respectively. In line with the FESEM observation, a higher magnification TEM image depicted in Fig. 3f indicates that the spheres are highly porous and composed of small nanocrystals with an average size of around 10–30 nm. In addition, the outer shell is very thin, with an average thickness of around 30 nm. A lattice spacing of 0.54 nm is observed in the high-resolution HRTEM image ( Supplementary Fig. 8 ), which is in good agreement with the interplanar spacing of NiCo 2 S 4 (111) planes. Elemental mapping based on energy-dispersive X-ray spectroscopy ( Supplementary Fig. 9 ) provides clearer information about the elemental distribution within the spheres. The distributions of Ni, Co and S elements in the hollow spheres are uniform, which further verifies the formation of phase-pure NiCo 2 S 4 . As determined by N 2 adsorption–desorption measurement ( Supplementary Fig. 10 ), these NiCo 2 S 4 ball-in-ball hollow spheres possess Brunauer–Emmett–Teller specific surface area of 53.9 m 2 g −1 . Besides, most of the pores are smaller than 10 nm in size, which are formed between the interconnected primary nanocrystals. 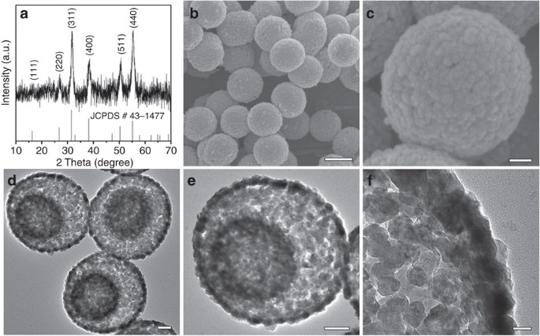Figure 3: Materials characterizations of the NiCo2S4ball-in-ball hollow spheres after annealing in N2. (a) XRD pattern, (b,c) FESEM images. Scale bars, 500 and 100 nm, respectively. (d,e) TEM images. Scale bars, 100 nm. (f) Enlarged TEM image of the NiCo2S4mesoporous shell. Scale bar, 20 nm. Figure 3: Materials characterizations of the NiCo 2 S 4 ball-in-ball hollow spheres after annealing in N 2 . ( a ) XRD pattern, ( b , c ) FESEM images. Scale bars, 500 and 100 nm, respectively. ( d , e ) TEM images. Scale bars, 100 nm. ( f ) Enlarged TEM image of the NiCo 2 S 4 mesoporous shell. Scale bar, 20 nm. Full size image More importantly, the present concept of structural design is facile and potentially represents a general strategy that can be used to synthesize other mixed metal sulfides with ball-in-ball architecture. As an example, uniform MnCo-glycerate spheres with a diameter of around 550 nm can be synthesized by a similar solvothermal method ( Supplementary Fig. 11a,b ). After the sulfidation reaction with TAA, the MnCo-glycerate precursor is chemically transformed into MnCo 2 S 4 ball-in-ball hollow spheres ( Supplementary Fig. 11c,d ). Electrochemical evaluation of ball-in-ball hollow spheres The pseudocapacitive properties of NiCo 2 S 4 ball-in-ball hollow spheres are evaluated by using a three-electrode cell configuration in 6.0 M KOH solution, and the results are shown in Fig. 4 . The representative cyclic voltammetry (CV) curves of the NiCo 2 S 4 electrode at various scan rates ranging from 2 to 60 mV s −1 in a potential window of −0.1 to 0.55 V are presented in Fig. 4a . The CV curves display two pairs of redox peaks, particularly at low scan rates, indicating the presence of redox reactions of NiCo 2 S 4 during the electrochemical process. With a 30-fold increment in the sweep rate, from 2 to 60 mV s −1 , there are no significant change in the position and shape of the current peaks, suggesting that the NiCo 2 S 4 electrode is favourable for fast redox reactions. 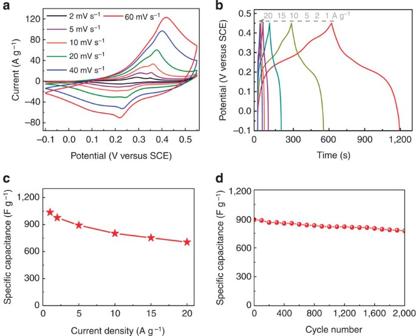Figure 4: Electrochemical characterizations of the NiCo2S4ball-in-ball hollow spheres electrode. (a) Cyclic voltammetry curves. (b) Galvanostatic charge/discharge voltage profiles. (c) Specific capacitance as a function of current density. (d) Cycling performance at a current density of 5 A g−1. SCE, saturated calomel electrode These distinct peaks might be attributed to the reversible Faradaic redox processes of Co 2+ /Co 3+ /Co 4+ and Ni 2+ /Ni 3+ redox couples based on the following reactions [40] , [43] : Figure 4: Electrochemical characterizations of the NiCo 2 S 4 ball-in-ball hollow spheres electrode. ( a ) Cyclic voltammetry curves. ( b ) Galvanostatic charge/discharge voltage profiles. ( c ) Specific capacitance as a function of current density. ( d ) Cycling performance at a current density of 5 A g −1 . SCE, saturated calomel electrode Full size image Figure 4b presents the galvanostatic charge/discharge curves of the NiCo 2 S 4 electrode at different current densities ranging from 1 to 20 A g −1 . Consistent with the CV results, the poorly defined voltage plateaus in the charge/discharge curves suggest the pseudocapacitive behaviour and the presence of some Faradaic processes. The specific capacitance of the NiCo 2 S 4 electrode as a function of current density, calculated from the discharge curves, is shown in Fig. 4c . A maximum specific capacitance reaches up to 1,036 F g −1 measured at a discharge current density of 1 A g −1 , and the corresponding volumetric capacitance is estimated to be 518 F cm −3 . With the increase of current density, the specific capacitance of the NiCo 2 S 4 electrode gradually decreases and still keeps a high value of 705 F g −1 at 20 A g −1 . About 68.1% of the capacitance for NiCo 2 S 4 ball-in-ball hollow spheres is retained when the current density increases from 1 to 20 A g −1 . Compared with NiCo 2 S 4 ball-in-ball hollow spheres, single-shelled NiCo 2 S 4 hollow spheres exhibit inferior electrochemical performance when characterized under similar conditions ( Supplementary Fig. 12 ), with a low specific capacitance of 567 F g −1 at 20 A g −1 , corresponding to around 57.7% of the capacitance at 1 A g −1 . The cycling performance of the NiCo 2 S 4 ball-in-ball hollow spheres electrode is evaluated by repeated charge/discharge test at a current density of 5 A g −1 . The specific capacitance is 892 F g −1 for the first cycle and the value decreases to 774 F g −1 with about 13% loss after continuous cycling for 2,000 cycles ( Fig. 4d ). After cycling, the hollow structure can be well retained but the primary nanoparticles change to nanosheets ( Supplementary Fig. 13 ). According to our previous experience, metal sulfides can be slowly electrochemically transformed into whisker-like metal hydroxides on the surface during the repeated charge/discharge processes [44] . Electrochemical evaluation of asymmetric capacitor To further evaluate the NiCo 2 S 4 electrode for practical application, an asymmetric supercapacitor (ASC) device is fabricated using the NiCo 2 S 4 electrode as the cathode and a nanocomposite graphene/carbon spheres (G/CSs) film electrode as the anode in KOH aqueous electrolyte, with one piece of cellulose paper as the separator ( Fig. 5a ). The flexible G/CS paper is fabricated by using a simple vacuum filtration method ( Supplementary Fig. 14 ). 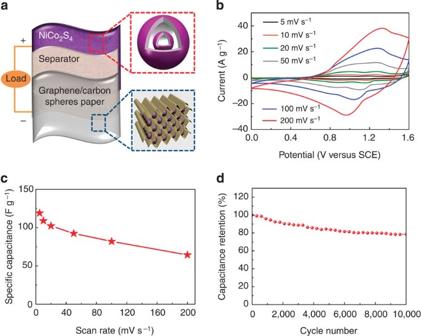Figure 5: Electrochemical evaluation of the NiCo2S4//G/CS ASC. (a) Schematic illustration of the ASC device. (b) CV curves of the ASC device at various scan rates from 5 to 200 mV s−1measured between 0 and 1.6 V. (c) Plot of the specific capacitance as a function of scan rate. (d) Cycling performance of the ASC device at a current density of 5 A g−1. SCE, saturated calomel electrode. Figure 5b presents typical CV curves of the NiCo 2 S 4 //G/CS ASC device at various scan rates between 0 and 1.6 V. Clearly, the CV curves show capacitance from both electric double-layer capacitance and pseudocapacitance. The current density increases with the increasing scan rate and all curves exhibit a similar shape. There is no obvious distortion in the CV curves even at a very high scan rate of 200 mV s −1 , indicating excellent fast-charge/discharge properties of the device. The calculated specific capacitance based on the CV curves as a function of the scan rate is plotted in Fig. 5c . The specific capacitance of the ASC is 119.1 F g −1 at the scan rate of 5 mV s −1 , and it still retains 64.3 F g −1 at a very high scan rate of 200 mV s −1 (based on the total mass of active materials of the two electrodes). Galvanostatic charge/discharge curves of the ASC at various current densities are shown in Supplementary Fig. 15 . The charge/discharge curves remain in a good symmetry at cell voltage as high as 1.6 V, implying that the cell has excellent electrochemical reversibility and capacitive characteristics. Figure 5d shows long-term cycling performance of the ASC at a current density of 5 A g −1 . Remarkably, the ASC manifests very high cycling stability and still delivers 78.6% of its initial capacitance even after 10,000 cycles. We have further evaluated the energy and power densities of the NiCo 2 S 4 //G/CS ASC. As shown in the Ragone plot ( Supplementary Fig. 16 ), the ASC displays a high energy density of 42.3 Wh kg −1 at a power density of 476 W kg −1 . Even at a high power density of 10208 W kg −1 , the ASC still delivers an energy density of 22.9 Wh kg −1 . Overall, the performance of this NiCo 2 S 4 //G/CS ASC is superior to that of many other ASCs, such as metal sulfide-based ASCs (CoS x //graphene [45] and Ni 3 S 2 //graphene [46] ), metal hydroxide-based ASCs (Ni(OH) 2 //activated carbon (AC) [47] ), metal oxide-based ASCs (NiO//graphene [48] and Co 3 O 4 //AC [49] ), mixed metal oxide-based ASCs (NiCo 2 O 4 //AC [50] and CoMoO 4 //AC [51] ). Figure 5: Electrochemical evaluation of the NiCo 2 S 4 //G/CS ASC. ( a ) Schematic illustration of the ASC device. ( b ) CV curves of the ASC device at various scan rates from 5 to 200 mV s −1 measured between 0 and 1.6 V. ( c ) Plot of the specific capacitance as a function of scan rate. ( d ) Cycling performance of the ASC device at a current density of 5 A g −1 . SCE, saturated calomel electrode. Full size image The pseudocapacitive properties of NiCo 2 S 4 ball-in-ball hollow spheres are compare favourably to or even superior to that of many binary or ternary nickel- and cobalt-based sulfides ( Supplementary Table 1 ) [36] , [37] , [38] , [39] , [40] , [41] , [43] , [52] , [53] , [54] , [55] , [56] , [57] . The improved pseudocapacitive performance of the NiCo 2 S 4 ball-in-ball hollow spheres might be largely attributed to their unique structure. First, the shells consisting of small nanocrystals possess high porosity, and thus the electrolyte can easily penetrate through the shell for efficient redox reactions during the Faradaic charge storage process. Second, the unique ball-in-ball hollow architecture could significantly enlarge the active surface area and probably improve the structural integrity as well. As a result, both the specific capacitance and cycling stability are greatly enhanced. In summary, a novel two-step method has been developed for the fabrication of NiCo 2 S 4 ball-in-ball hollow spheres with enhanced pseudocapacitive properties. The synthesis involves a facile solvothermal synthesis of uniform NiCo-glycerate solid spheres and a subsequent chemical sulfidation process. The formation mechanism of such interesting ball-in-ball hollow structures could be attributed to the discrepancy in diffusion rates of metal cations and sulfide anions during the sulfidation process. The resultant NiCo 2 S 4 ball-in-ball hollow spheres exhibit a high specific capacitance of 1,036 F g −1 at a current density of 1.0 A g −1 . An asymmetric supercapacitor has been successfully fabricated using these unique NiCo 2 S 4 hollow spheres, which delivers high energy and power densities and exhibits outstanding cycle life. This work would open up new strategies for the controllable synthesis of complex hollow structures of metal sulfides and other functional materials for different applications. Synthesis of NiCo 2 S 4 ball-in-ball hollow spheres All the chemicals were directly used after purchase without further purification. In a typical synthesis, 0.25 mmol of Co(NO 3 ) 2 ·6H 2 O, 0.125 mmol of Ni(NO 3 ) 2 ·6H 2 O and 8 ml of glycerol were dissolved into 40 ml of isopropanol to form a transparent pink solution. The solution was then transferred to a Teflon-lined stainless steel autoclave and kept at 180 °C for 6 h. After cooling to room temperature naturally, the brown precipitate was separated by centrifugation, washed several times with ethanol and dried in an oven at 80 °C. For the preparation of NiCo 2 S 4 hollow spheres, 30 mg of the above NiCo-glycerate precursor was re-dispersed into 20 ml of ethanol, followed by the addition of 50 mg of TAA. Then the mixture was transferred into a Teflon-lined stainless steel autoclave and kept at different temperature. After centrifugation and washed with ethanol for several times, the NiCo 2 S 4 hollow spheres were obtained. To improve the crystallinity, the final product was annealed under N 2 atmosphere at 300 °C for 0.5 h. Synthesis of G/CS paper Ordered mesoporous CSs were prepared by a hydrothermal method reported by Zhao et al . [58] The freshly prepared carbon spheres were functionalized with poly(diallyldimethylammonium chloride) to own surface positive charges. Graphene oxide (GO) was synthesized from natural graphite flakes by a modified Hummers method [59] . The G/CS paper was prepared by the following process: GO (30 mg) was dispersed in distilled water (40 ml) by ultrasonic treatment for 2 h. CS functionalized with poly(diallyldimethylammonium chloride) (6 mg) were added and then sonicated for another 2 h. The resulting complex dispersion was filtered by a vacuum filter equipped with a 0.2-μm porous polytetrafluoroethylene membrane to produce a GO/CS paper. Subsequently, hydrazine in gas form was applied in a reaction chamber under ambient conditions for 3 days to reduce the GO to form G/CS paper. Materials characterization Powder XRD patterns were collected on a Bruker D2 Phaser X-Ray Diffractometer with Ni filtered Cu Kα radiation ( λ =1.5406 Å) at a voltage of 30 kV and a current of 10 mA. The microstructures were characterized using TEM (JEOL, JEM-2010) and FESEM (JEOL, JSM-6700F). Elemental mapping was acquired using energy-dispersive X-ray spectroscopy attached to JEM-2100F (TEM, JEOL). The N 2 sorption measurement was carried on Autosorb 6B at liquid N 2 temperature. Electrochemical measurements For electrochemical measurements, the working electrode was prepared by mixing the electroactive material, carbon black (super-P-Li) and polymer binder (polyvinylidene difluoride) in a weight ratio of 70:20:10. The slurry was pressed onto Ni foam and dried at 90 °C for 10 h. Electrochemical measurements were conducted with a CHI 660C electrochemical workstation in an aqueous KOH electrolyte (6.0 M) with a three-electrode cell where a Pt foil serves as the counter electrode and a saturated calomel electrode as the reference electrode. The tap density of the NiCo 2 S 4 ball-in-ball hollow spheres was estimated by directly measuring the mass and physical dimensions occupied, which is about 0.5 g cm −3 . The mass loading of NiCo 2 S 4 is about 5 mg cm −2 . The specific capacitance is calculated by the following equation: where I is the discharge current, Δ t is the discharge time, Δ V is the voltage range and m is the mass of the active material. The volumetric capacitance is calculated by the following equation: where C v is the volumetric capacitance, C m is the gravimetric capacitance and ρ is the materials density. Fabrication and evaluation of supercapacitor devices ASCs were fabricated by assembling NiCo 2 S 4 cathode and graphene/CS anode with one piece of cellulose paper as the separator in two-electrode simulation cells. A 6 M KOH solution was employed as the electrolyte. The mass ratio of positive electrode to negative electrode was decided according to the well-known charge balance equation ( q + = q − ). In the relation, the charge stored by each electrode usually depends on the specific capacitance ( C ), the potential range (Δ V ) and the mass of the electrode ( m ) following equation (6): To obtain q + = q − , the mass balance will be expressed as following equation (7): C + and C − are the specific capacitance of the NiCo 2 S 4 and G/CS electrodes, respectively. Δ V + and Δ V − are the voltage range of one scanning segment (V) of NiCo 2 S 4 and G/CS electrodes, respectively. The specific capacitance ( C ) is calculated from the CV curve by following Equation 8: where I is the current density (A cm −2 ), V is the cell voltage (V), v is the potential scan rate (mV s −1 ) and m is the total mass of active materials on both electrodes (g cm −2 ). The energy density ( E ) and power density ( P ) of ASCs against the two electrodes in device were calculated based on the total mass of the active materials using the following equations: where V is the voltage range of one sweep segment and Δ t is the time for a sweep segment. How to cite this article : Shen, L. et al . Formation of nickel cobalt sulfide ball-in-ball hollow spheres with enhanced electrochemical pseudocapacitive properties. Nat. Commun. 6:6694 doi: 10.1038/ncomms7694 (2015).